Insight into spin transport in oxide heterostructures from interface-resolved magnetic mapping At interfaces between complex oxides, electronic, orbital and magnetic reconstructions may produce states of matter absent from the materials involved, offering novel possibilities for electronic and spintronic devices. Here we show that magnetic reconstruction has a strong influence on the interfacial spin selectivity, a key parameter controlling spin transport in magnetic tunnel junctions. In epitaxial heterostructures combining layers of antiferromagnetic LaFeO 3 (LFO) and ferromagnetic La 0.7 Sr 0.3 MnO 3 (LSMO), we find that a net magnetic moment is induced in the first few unit planes of LFO near the interface with LSMO. Using X-ray photoemission electron microscopy, we show that the ferromagnetic domain structure of the manganite electrodes is imprinted into the antiferromagnetic tunnel barrier, endowing it with spin selectivity. Finally, we find that the spin arrangement resulting from coexisting ferromagnetic and antiferromagnetic interactions strongly influences the tunnel magnetoresistance of LSMO/LFO/LSMO junctions through competing spin-polarization and spin-filtering effects. The recent years have seen the discovery of various examples of emerging phenomena at oxide interfaces [1] , [2] , [3] , [4] , [5] , broadening the scope of oxide electronics [6] . Some already offer novel device opportunities, as demonstrated for several systems [7] , [8] , [9] , [10] , [11] . In the context of spintronics, magnetic reconstruction at the interface between a ferromagnetic oxide and a nonferromagnetic oxide [12] , [13] , [14] can enrich the physics of spin transport in magnetic tunnel junctions (MTJs) [15] , [16] . For instance, induced magnetic moments due to super-exchange interaction across interfacially reconstructed chemical bonds [17] have been proposed to give rise to an induced magnetic state at the barrier, with deep consequences for tunnel transport due to spin (de)polarization [8] . Beyond an exotic spin transport response, the presence of magnetic moments in the barrier material can also influence magnetic switching and produce complex micromagnetic behaviour [8] , [18] , [19] , [20] . To date, the existence of induced ferromagnetic domains in an otherwise nonferromagnetic barrier has, however, not been proven. For that, conventional sample averaging methods such as superconducting quantum interference device (SQUID) or Kerr magnetometry or magnetic spectroscopies with in-depth spatial resolution such as polarized neutron reflectometry, must be supplemented by element-specific and magnetic-sensitive X-ray magnetic circular dichroism (XMCD) combined with microscopy techniques such as photoemission electron microscopy (PEEM) [21] with lateral spatial resolution. Here we report a ferromagnetic domain state induced into an antiferromagnetic barrier at the interface between La 0.7 Sr 0.3 MnO 3 (LSMO) and LaFeO 3 (LFO). We study multilayers and MTJs combining LSMO (a half-metallic ferromagnet with a high Curie temperature T C =350 K (refs 22 , 23 )) and LFO (an antiferromagnetic insulator with a Néel temperature of 740 K (ref. 24 )). By means of X-ray PEEM, we collect maps of the magnetic domains as a function of magnetic field in the top and bottom electrodes of a LSMO/LFO/LSMO tunnel junction, and correlate them with tunnel magnetoresistance (TMR) cycles. We show that the magnetic domain state of the electrodes is imprinted into the barrier, giving rise to strong modifications of the tunnelling transport due to emerging spin filtering by the imprinted ferromagnetic state. These results bring key insights into the dependence of the junction resistance as a function of field, bias and temperature, and suggest routes for the optimal combination of electrode and barrier effects in spin transport. Oxide heterostructure samples We have grown a series of [LSMO N /LFO M ] heterostructures, where N and M denote the nominal thickness in nanometres of each layer. All samples were synthesized on (001)-oriented SrTiO 3 substrates by high pressure pure oxygen sputtering deposition. For structural characterization, we used superlattices consisting of six bilayers of LSMO/LFO. LSMO/LFO (LFO top ) and LFO/LSMO (LFO bot ) interfaces were studied in bilayers with the LFO on top of the LSMO ((LSMO 35 /LFO 1.2 ) bilayer) or below the LSMO ((LFO 1.2 /LSMO 3.5 ) bilayer), respectively. In these samples, we used a reduced LFO thickness (1.2 nm, that is, three unit cells) so that the spectroscopic signal in LFO is dominated by the interface. Finally (LSMO 35 /LFO 3.5 /LSMO 8 ) stacks were patterned into MTJs by optical lithography to perform magnetotransport measurements and study magnetic domains by XMCD–PEEM in device geometry. 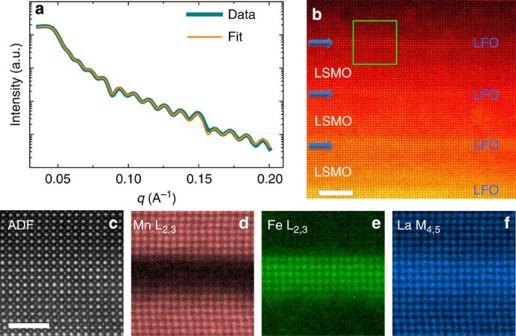Figure 1: Structural characterization. (a) X-ray reflectivity spectrum (blue) and fit (orange) of a (LSMO5.9/LFO2.7)X6superlattice. (b) High resolution Z-contrast scanning transmission electron microscopy image of the same sample. The labels and arrows indicate the LFO and LSMO layers in the superlattice. The green box marks the area where the elemental maps were obtained. The scale bar, 5 nm. (c) Annular dark field (ADF) signal acquired simultaneously with the EEL spectrum image. Minor spatial drift is observed. The scale bar, 2 nm. Atomic resolution elemental maps obtained from the analysis of the (d) Mn L3,2, (e) Fe L3,2and (f) La M4,5edges. Structural characterization Figure 1a shows X-ray reflectivity (XRR) data (blue) for a (LSMO 5.9 /LFO 2.7 ) x6 superlattice. The presence of high-order superlattice and finite thickness oscillations confirms the high quality of the interfaces over long lateral distances. The thickness determined from a fit [25] (orange curve) to the data was 6 nm for LSMO and 2.6 nm for LFO, in close agreement with the nominal layer thickness. The roughness is 0.4 nm for the LSMO on LFO interface and 0.2 nm for LFO on LSMO. Figure 1: Structural characterization. ( a ) X-ray reflectivity spectrum (blue) and fit (orange) of a (LSMO 5.9 /LFO 2.7 ) X6 superlattice. ( b ) High resolution Z-contrast scanning transmission electron microscopy image of the same sample. The labels and arrows indicate the LFO and LSMO layers in the superlattice. The green box marks the area where the elemental maps were obtained. The scale bar, 5 nm. ( c ) Annular dark field (ADF) signal acquired simultaneously with the EEL spectrum image. Minor spatial drift is observed. The scale bar, 2 nm. Atomic resolution elemental maps obtained from the analysis of the ( d ) Mn L 3,2 , ( e ) Fe L 3,2 and ( f ) La M 4,5 edges. Full size image To further characterize the interface quality of the same sample, we used scanning transmission electron microscopy (STEM). In the high angle annular dark field (ADF) image shown in Fig. 1b , the contrast between the layers is related to the atomic number of the atoms, hence the difficulties to distinguish the LSMO and LFO layers. To better study the interface structure, we have acquired elemental maps in the area marked in Fig. 1b using electron energy loss spectroscopy (EELS). The simultaneously acquired ADF image as well as the elemental maps corresponding to the Mn L 3,2 , Fe L 3,2 and La M 4,5 absorption edges are shown in Fig. 1c–f . The LFO and LSMO layers are clearly resolved when comparing Fig. 1d,e and together with the ADF images prove the good epitaxial properties and coherent growth of these materials. Induced moment in LFO To gain insight into the electronic and magnetic structure of the LFO top interface, we performed X-ray absorption spectroscopy (XAS) experiments using the Alice chamber at the PM3 beamline of the Helmholtz-Zentrum-Berlin (HZB). The fluorescence yield absorption spectra measured in a (LFO 1.2 /LSMO 3.5 ) bilayer at Mn L 3,2 and Fe L 3,2 edges and 60 K are displayed in Fig. 2a,d (solid line), respectively. The spectra agree well with those previously reported for these materials [26] , confirming the expected 3+/4+ Mn mixed valence in LSMO and dominant Fe 3+ character in LFO. In Fig. 2d , we also show a simulated spectrum (dashed line) for pure Fe 3+ based on charge-transfer multiplet calculations obtained with CTM4XAS [27] . A good agreement with the data is obtained using a crystal field with fourfold symmetry (C 4 ) with a value of 10 Dq=1.8 eV for Fe 3+ (ref. 26 ). 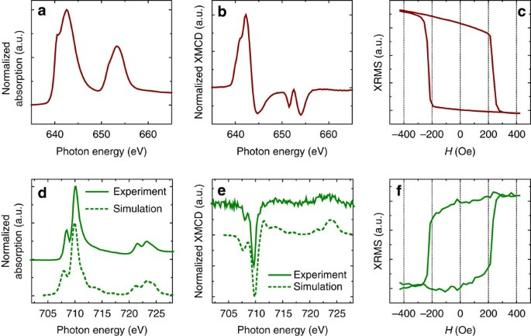Figure 2:Induced moment in LaFeO3. Measured (solid lines) and simulated (dashed lines) X-ray absorption (a,d) and X-ray magnetic circular dichroism (b,e) spectra obtained at 60 K in a (LFO1.2/LSMO3.5) heterostructure. The spectra were obtained at the Mn L3,2(a,b) and Fe L3,2(d,e) edges. X-Ray resonant magnetic scattering (XRMS) as a function of magnetic field obtained with photon energies (c)E=642.2 eV, Mn L3,2edge and (f)E=709.7 eV, Fe L3,2edge. Figure 2: Induced moment in LaFeO 3 . Measured (solid lines) and simulated (dashed lines) X-ray absorption ( a , d ) and X-ray magnetic circular dichroism ( b , e ) spectra obtained at 60 K in a (LFO 1.2 /LSMO 3.5 ) heterostructure. The spectra were obtained at the Mn L 3,2 ( a , b ) and Fe L 3,2 ( d , e ) edges. X-Ray resonant magnetic scattering (XRMS) as a function of magnetic field obtained with photon energies ( c ) E =642.2 eV, Mn L 3,2 edge and ( f ) E =709.7 eV, Fe L 3,2 edge. Full size image The difference between XAS spectra measured with left- and right-circular-polarized light yields element-specific magnetic information. Equivalently, here we fix the light helicity and measure XAS for two opposite magnetization directions. Figure 2b shows the XMCD signal measured for the LSMO layers [14] , [28] , [29] . At the Fe L 3,2 edge ( Fig. 2e , solid line), a nonzero XMCD signal is detected, indicating the presence of a net magnetic moment in the nominally antiferromagnetic LFO layer. A similar XMCD spectrum was previously observed in the related compound GaFeO 3 , known to be ferrimagnetic, and was ascribed to magnetism in pure Fe 3+ (ref. 30 ). Here we were able to simulate the XMCD signal by simply adding an exchange field to the crystal environment of the Fe 3+ atom. Again, the simulations (dashed line in Fig. 2e ) reproduce well the data, which further confirms the dominant 3+ character of the Fe ions. The energy dependence of the Mn and Fe XMCD shows that the net magnetic moment in LSMO and LFO are antiparallel to each other. The net magnetic moment of the Fe atom obtained by applying sum rules is 0.03 μ B /Fe (ref. 31 ). This value should be taken as a lower limit to the magnetic moment since the measurement is normalized to the 1.2 nm thickness of the LFO layer; supposing that only the FeO 2 plane closest to the interface acquires a magnetic moment yields 0.09 μ B /Fe. It is known that a nonferromagnetic material may acquire a net magnetic moment at the interface with a ferromagnet in epitaxial oxide heterostructures. Examples include the measured magnetic moment at the Cu L 3,2 edge in La 0.7 Ca 0.3 MnO 3 /YBa 2 Cu 3 O 7 (refs 12 , 32 ) or La 0.7 Ca 0.3 MnO 3 /PrBa 2 Cu 3 O 7 interfaces [33] and at the Ti L-edge in manganite/SrTiO 3 interfaces [4] , [14] , [34] . In both cases the magnetic moment is explained by a coupling between the Mn and the corresponding transition metal ion (that is, Cu or Ti) at the interface. A Mn–Fe coupling scenario fits with our observations and is indeed confirmed by collecting element-specific hysteresis loops at the Mn and Fe L 3,2 edges. Figure 2c,f present such loops measured by means of X-ray resonant magnetic scattering. The coercive and saturation fields in both cycles coincide, confirming the strong (antiferro)magnetic coupling between the Mn and Fe moments. With the aim of studying the micromagnetics of the LFO bot and LFO top interfaces in MTJs, we have performed XMCD–PEEM experiments on (LSMO 35 /LFO 1.2 ) and (LSMO 35 /LFO 3.5 /LSMO 8 ) samples patterned into 8.5 × 2.8 μm mesa structures, respectively (see sketch in Fig. 3e,f ). XMCD–PEEM images were obtained at both Mn and Fe L 3 edges. 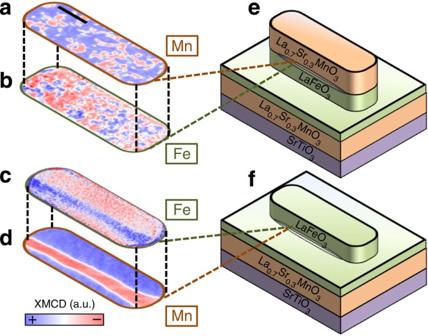Figure 3: Magnetic mapping at interfaces. XMCD–PEEM images obtained with photon energies (a,d)E=642.2 eV (Mn L3,2edge) and (b,c)E=709.7 eV (Fe L3,2edge). (e) Schematic of a patterned (LSMO35/LFO3.5/LSMO8) heterostructure where the (a,b) images were obtained. (f) Schematic of a patterned (LSMO35/LFO1.2) heterostructure where the (c,d) images were obtained. The XMCD colour scale is proportional to the magnetic moment along the long axis of the patterned junction and is normalized to a fully saturated state to either Fe or Mn XMCD signal. Notice that at each interface the magnetic domains in the LSMO layer are imprinted into the LFO layer through Fe–Mn antiferromagnetic coupling. A 2 μm scale bar is shown ina: the scale is the same for all PEEM images. Figure 3a–d shows the magnetic domain structure for the LFO top (LFO bot ) interface at 120 K. Magnetic domains are clearly resolved in both LSMO ( Fig. 3a,d ) and LFO layers ( Fig. 3b,c ). There is a one-to-one correlation between LSMO and LFO domains at each interface. Note, however, that they show an opposite red–blue contrast highlighting their antiparallel alignment. We conclude that the LSMO domains are magnetically imprinted into the LFO layers through the antiferromagnetic Fe–Mn alignment observed in the XMCD data, see Fig. 2 . Note that the uncompensated Fe moments did not produce exchange bias shifts in M ( H ) loops measured at low temperature after cooling in 1 T, possibly owing to the small thickness of the antiferromagnet [35] . Figure 3: Magnetic mapping at interfaces. XMCD–PEEM images obtained with photon energies ( a , d ) E =642.2 eV (Mn L 3,2 edge) and ( b , c ) E =709.7 eV (Fe L 3,2 edge). ( e ) Schematic of a patterned (LSMO 35 /LFO 3.5 /LSMO 8 ) heterostructure where the ( a , b ) images were obtained. ( f ) Schematic of a patterned (LSMO 35 /LFO 1.2 ) heterostructure where the ( c , d ) images were obtained. The XMCD colour scale is proportional to the magnetic moment along the long axis of the patterned junction and is normalized to a fully saturated state to either Fe or Mn XMCD signal. Notice that at each interface the magnetic domains in the LSMO layer are imprinted into the LFO layer through Fe–Mn antiferromagnetic coupling. A 2 μm scale bar is shown in a : the scale is the same for all PEEM images. Full size image In operando magnetic mapping of LSMO/LFO/LSMO junctions Next, we collected XMCD–PEEM images at the Mn L 3 edge for a patterned junction at 120 K during a magnetic field sweep (from about 400 to −400 Oe and back), see Fig. 4a–n . Domains observed in the junction area correspond to the top electrode, whereas domains outside the junction give information on the nonpatterned bottom electrode. We have analyzed the images and calculated the integrated XMCD–PEEM signal (proportional to the magnetization) for the top electrode and the surrounding area. From the integrated XMCD, we extracted for both electrodes the relative contribution of domains with a positive magnetization ( F top and F bot ), which we plot below the images ( Fig. 4o,p ). 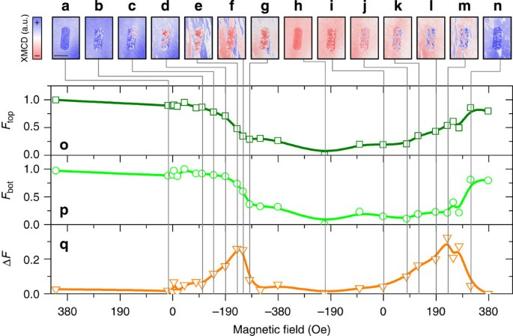Figure 4: Magnetic field dependence of magnetic domains in a LSMO/LFO/LSMO tunnel junction. (a–n) XMCD–PEEM images measured atE=642.2 eV, Mn L3,2edge. The images were obtained while sweeping the magnetic field from 380 to −380 Oe and back to 380 Oe on (LSMO35/LFO3.5/LSMO8) heterostructure patterned into a MTJ. The magnetic field was applied along the long axis of the junctions, the colour scale is proportional to the magnetic moment along this direction and is normalized to the Mn XMCD signal in a fully saturated state. Positive fraction of the integrated XMCD signal in the top (Ftop,o) and the bottom (Fbot,p) electrodes as a function of magnetic field. ΔF=|Ftop−Fbot| is plotted against the magnetic field inq. Lines are B-splines passing through the data. The grey lines are guides to the eyes and indicate the magnetic field at which each image was measured. A 5 μm scale bar is shown ina: the scale is the same for all PEEM images. Figure 4q shows the fraction of regions having a positive contribution to the XMCD signal in one but not the other electrode, that is, Δ F =| F top − F bot |. Figure 4: Magnetic field dependence of magnetic domains in a LSMO/LFO/LSMO tunnel junction. ( a – n ) XMCD–PEEM images measured at E =642.2 eV, Mn L 3,2 edge. The images were obtained while sweeping the magnetic field from 380 to −380 Oe and back to 380 Oe on (LSMO 35 /LFO 3.5 /LSMO 8 ) heterostructure patterned into a MTJ. The magnetic field was applied along the long axis of the junctions, the colour scale is proportional to the magnetic moment along this direction and is normalized to the Mn XMCD signal in a fully saturated state. Positive fraction of the integrated XMCD signal in the top ( F top , o ) and the bottom ( F bot , p ) electrodes as a function of magnetic field. Δ F =| F top − F bot | is plotted against the magnetic field in q . Lines are B-splines passing through the data. The grey lines are guides to the eyes and indicate the magnetic field at which each image was measured. A 5 μm scale bar is shown in a : the scale is the same for all PEEM images. Full size image In Fig. 4a taken near magnetic remanence after saturating the sample in a positive field, the electrodes present an homogeneous magnetization in the top and bottom layers and F top and F bot are both close to 1, as expected. As the field is swept towards large negative values, domains with reversed orientation start to nucleate in the top electrode ( Fig. 4b ) and then grow in size ( Fig. 4c ). In this range, F bot stays constant but F top starts to decrease. In Fig. 4d , the nucleation of domains in the bottom electrode has begun. Reversed domains in both electrodes then develop ( Fig. 4e,f ) and both F top and F bot strongly decrease. Magnetization reversal is almost complete in Fig. 4g . Figure 4h is taken after saturation in a negative field and both F top and F bot are close to 0. When the field is swept in the opposite direction, a similar process is observed ( Fig. 4i–n ). Again, reversal starts at weaker fields for the top electrode and is sharper in the bottom layer. A first observation derived from the magnetic domain mapping is that the shape of the domains is different in both layers. While in the bottom layer, domains are stripe-shaped and larger, in the top layer the domains are smaller, more irregular and form a mosaic pattern. The different domain size and shape might be related to the different thicknesses of the manganite layers [36] . Second, a situation in which the top and bottom electrodes have a homogeneous magnetization with an antiparallel alignment is never reached. Figure 4q indicates that at most ~30% of domains have opposite magnetization directions (that is, are antiparallel to each other) near ±230 Oe. (LSMO 35 /LFO 3.5 /LSMO 8 ) heterostructures similar to those imaged by XMCD–PEEM were patterned into MTJs, and Fig. 5a shows a typical R versus H measurement at a bias voltage of 1 mV and T =100 K. As the field is swept from H =400 to −400 Oe, the MTJ transitions from a low resistance parallel state ( R low ) to a high resistance antiparallel state ( R high ) near −200 Oe. On increasing the field further, the resistance switches back to R low at approximately −300 Oe. For this junction, the tunnelling magnetoresistance calculated here as TMR=( R high − R low )/ R low reaches ~30%, a moderate TMR value compared with other full-oxide manganite-based tunnel junctions [8] , [37] , [38] . To evaluate how the electrodes’ micromagnetism is responsible for this low value, we have computed the TMR value expected from the magnetic switching behaviour presented in Fig. 4 (within Jullière’s model [39] ). We assume tunnel conduction in parallel between parallel (red-to-red or blue-to-blue in the XMCD–PEEM images) or antiparallel (red-to-blue or blue-to-red) domains. We have only indirect information on the bottom electrode domain configuration (from that of its surroundings), but because the micromagnetism of both electrodes is very different we assume no coupling between them, and that the LSMO in the bottom electrode under the top one behaves on average as that in the surroundings. We thus use Δ F as the relative fraction of antiparallel domains. Then, we apply Jullière’s model [39] taking an average spin-polarization value (for top and bottom electrode) P =0.75 for LSMO [38] . The results are plotted in Fig. 5b . The global shape of the calculated TMR curve resembles that of the experimental one ( Fig. 5a ), and the maximum calculated TMR is ~30%, in good agreement with the experiments. This indicates that the rather low TMR value is largely due to the micromagnetics of the junctions and the inability to achieve >30% of antiparallel domains. 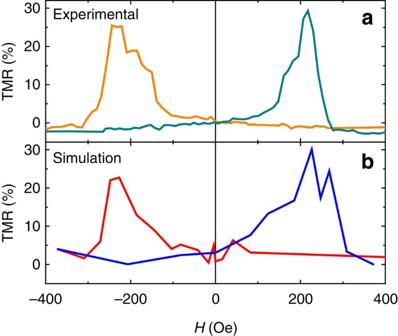Figure 5: Tunnel magnetoresistance. Tunnelling magnetoresistance in a (LSMO35/LFO3.5/LSMO8) junction obtained while sweeping the magnetic field from positive to negative values (orange and red lines) and back (cyan and blue lines) (a) Experimental dependence of the TMR measured with a 1 mV bias atT=100 K. (b) Simulated TMR using the Jullière’s model and the magnetic configuration experimentally obtained from XMCD–PEEM images. Figure 5: Tunnel magnetoresistance. Tunnelling magnetoresistance in a (LSMO 35 /LFO 3.5 /LSMO 8 ) junction obtained while sweeping the magnetic field from positive to negative values (orange and red lines) and back (cyan and blue lines) ( a ) Experimental dependence of the TMR measured with a 1 mV bias at T =100 K. ( b ) Simulated TMR using the Jullière’s model and the magnetic configuration experimentally obtained from XMCD–PEEM images. Full size image Temperature dependence of the magnetic and spintronic response We now turn to the influence of temperature on the magnetic and spintronic response. In Fig. 6a,b , we show the temperature dependence of the XMCD signals measured at remanence and in fluorescence yield for the (LFO 1.2 /LSMO 3.5 ) heterostructure, together with that of the magnetization ( Fig. 6c ). In this sample, the Curie temperature is ~210 K, and the XMCD signal at the Mn L 3,2 edge disappears a few tens of K lower ( T C-Mn ≈185 K), possibly reflecting the well-known depression of magnetic properties at interfaces and surfaces of manganites [22] , [40] . 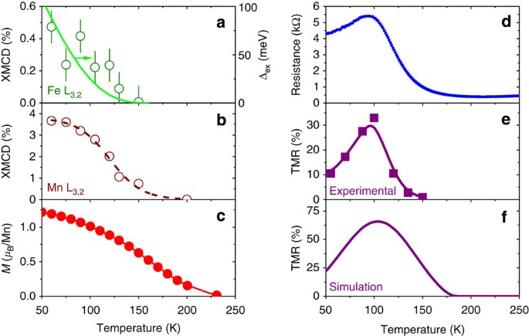Figure 6: Temperature dependence of the magnetic and spintronic response. (a) Temperature dependence of the XMCD at the Fe L3,2edge (left axis) and of the exchange splitting in the LFO barrier used to compute the curve inf(right axis). (b) Temperature dependence of the XMCD at the Mn L3,2edge (the dotted line is a guide to the eye). (c) Magnetization versus temperature obtained in (LFO1.2/LSMO3.5). (d) Temperature dependence of the junction resistance. Temperature dependence of the TMR: (e) experimental (the line is a B-spline passing through the data), (f) simulations. The XMCD signal at the Fe L 3,2 edge globally follows the same trend and vanishes near T C–Fe ≈150 K. Figure 6: Temperature dependence of the magnetic and spintronic response. ( a ) Temperature dependence of the XMCD at the Fe L 3,2 edge (left axis) and of the exchange splitting in the LFO barrier used to compute the curve in f (right axis). ( b ) Temperature dependence of the XMCD at the Mn L 3,2 edge (the dotted line is a guide to the eye). ( c ) Magnetization versus temperature obtained in (LFO 1.2 /LSMO 3.5 ). ( d ) Temperature dependence of the junction resistance. Temperature dependence of the TMR: ( e ) experimental (the line is a B-spline passing through the data), ( f ) simulations. Full size image Let us now address how the induced moment in the LFO layer influences spin transport in LSMO/LFO/LSMO MTJs. Figure 6d displays the temperature dependence of the junction resistance. On cooling, the resistance starts to increase, shows a maximum near 100 K and then decreases. This behaviour is anomalous compared with that of conventional MTJs but is found in tunnel junctions with ferromagnetic barriers, that is, in spin filters [41] . Below the Curie temperature of the ferromagnetic barrier, exchange splitting effectively reduces the tunnel barrier height for one type of carriers, which decreases the junction resistance [42] . As visible in Fig. 6e , the evolution with temperature of the TMR is also anomalous: on decreasing the temperature, a TMR signal of ~1% appears at 150 K and continues to rise up to ~33% at 100 K. Surprisingly, the TMR then decreases to ~8% only at 25 K. This dependence is in stark contrast with the monotonic increase of TMR with decreasing temperature that is usually found in manganite-based junctions, due to the increase of the electrodes’ spin polarization as temperature is lowered [38] . We argue here that the presence of an induced magnetic moment in the LFO (inferred from the XMCD and PEEM data) exchange splits the band structure of the material. When used as a tunnel barrier, this results in different transmission coefficients for spin-up and spin-down electrons, that is, spin filtering. This effect starts to occur when the LFO develops a magnetic moment, that is a few tens of K below the T C of the LSMO electrodes. Generally, depending on the sign of the exchange splitting 2Δ ex in the barrier with respect to that in the electrodes, spin filtering can either amplify the positive spin-polarization of electrons tunnelling from the adjacent LSMO electrode, reduce it or change its sign. Here because the sign of the net magnetic moment induced in LFO is opposite to that in LSMO, one of the latter two scenarios must be true (small or large Δ ex limit, respectively). In this scenario, we can model the temperature dependence of the TMR following the study by Liu et al. [15] At each LSMO/LFO interface, we consider that LFO is ferromagnetic over d =3 unit cells, with a spin-split density of states. In the Wenzel–Kramer–Brillouin (WKB) approximation, we compute the transmission of spin-up and spin-down electrons, deduce the tunnelling conductance in the parallel and antiparallel magnetization states ( G p and G ap , respectively) and the TMR=( G p − G ap )/ G ap (see Methods for more details). To compute the temperature dependence of the TMR, we assume that Δ ex is proportional to the magnetic moment [42] in the LFO layer, with a Curie point near 150 K (see the plot in Fig. 6a , right axis). Above this temperature, the dependence of the TMR will be largely determined by the behaviour of the top electrode, which owing to its lower thickness (8 nm) has a lower T C than the thicker bottom electrode (35 nm). The interfacial spin polarization of LSMO is known to decay faster than the magnetization [22] , [38] , and for this 8 nm electrode its temperature dependence likely resembles that of the XMCD Mn signal of the (LFO 1.2 /LSMO 3.5 ) sample plotted in Fig. 6b . The results of this simulation are plotted in Fig. 6f . The calculated curve reproduces well the global shape of the experimental data, that is, an increase of the TMR with temperature at low temperature, a maximum near 100 K and a decrease beyond this temperature. The maximum calculated TMR is ~65% compared with 32% for the data, and this difference can be largely ascribed to the micromagnetism of the junctions, as discussed previously. Note that here we do not take into account spin-depolarizing inelastic effects, such as magnon excitations by the tunnelling electrons [43] , [44] (that would increasingly reduce the TMR as temperature is lowered below ~100 K), or exchange interactions between the tunnelling spins and the paramagnetic moments in the barrier [45] (that would cause a stronger decrease of the TMR beyond the Curie point of the LFO). To further confirm that spin filtering is at play in our junctions, we look for its specific signatures [8] , [46] in the bias ( V ) dependence of the TMR. 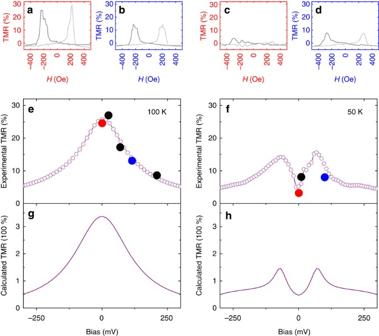Figure 7: Bias voltage dependence of the tunnel magnetoresistance. Resistance as a function of the magnetic field obtained at (a) 100 K and 1 mV, (b) 100 K and 100 mV, (c) 50 K and 1 mV and (d) 50 K and 100 mV bias. TMR as a function of bias measured at (e) 100 K and (f) 50 K. Data in open symbols were obtained fromI(V) curves and those in solid symbols fromR(H) curves (including those shown ina–d; the colour of the graph frame ina–dcorresponds to that of the symbol ine,f). Simulations of the bias dependence of the TMR at 100 K (g) and 50 K (h). Figure 7e,f shows the TMR( V ) at 100 K and 50 K, respectively, that is, near the barrier’s T C or well into the barrier’s ferromagnetic-like regime. Figure 7a–d presents examples of R ( H ) curves measured at different biases and temperatures. The bias dependence of the TMR observed at T =100 K follows the usual behaviour [47] , with the TMR decreasing for increasing bias. At T =50 K, however, the TMR increases with increasing voltage up to ~70 mV and then decreases as bias increases further. This is the behaviour expected for spin filters [8] , [46] . Indeed, as bias voltage is increased a transition from direct tunnelling to Fowler–Nordheim tunnelling occurs earlier for electrons of one spin type than for the other. Tunnel transmission is then strongly favoured for one spin direction compared with the other and near that point at which the TMR reaches a maximum value [48] , [49] . Beyond, the TMR decreases as in classical MTJs. Figure 7: Bias voltage dependence of the tunnel magnetoresistance. Resistance as a function of the magnetic field obtained at ( a ) 100 K and 1 mV, ( b ) 100 K and 100 mV, ( c ) 50 K and 1 mV and ( d ) 50 K and 100 mV bias. TMR as a function of bias measured at ( e ) 100 K and ( f ) 50 K. Data in open symbols were obtained from I ( V ) curves and those in solid symbols from R ( H ) curves (including those shown in a – d ; the colour of the graph frame in a – d corresponds to that of the symbol in e , f ). Simulations of the bias dependence of the TMR at 100 K ( g ) and 50 K ( h ). Full size image Figure 7g,h are simulations of the TMR( V ) at 100 K and using the same barrier parameters as for Fig. 6f . Data were interpreted in the framework of a WKB electron tunnelling, which yields a barrier height of 0.25 eV. This value is considerably smaller than the ~1.5 eV expected from the differences in electron affinity of LFO (3.3 eV) and the work function of LSMO (4.8 eV). However, this discrepancy can be resolved by assuming a few per cent electron-doping of the LFO interfaces (possibly resulting from the presence of oxygen vacancies), undetected by our XAS measurements. In addition, we also take into account spin-depolarizing inelastic effects through a phenomenological Lorentzian decay of the tunnelling electron spin-polarization [50] . For both sets of data, the simulations reproduce well the experiments, notably the nonmonotonous TMR( V ) at 50 K (note that again the calculated TMR maximum amplitude is larger due to micromagnetic effects). This brings further evidence that the transport response of the junctions is determined by a competition between the large spin-polarization of the electrodes, spin-filtering effects in the barrier and spin-depolarizing mechanisms in both the electrodes and the barrier. In summary, we have shown that the novel magnetic phases that arise at interfaces profoundly modify the behaviour of spintronic architectures based on complex oxide devices (here LSMO/LFO/LSMO tunnel junctions). Using XMCD–PEEM images obtained with an applied magnetic field while switching an MTJ, we have brought insights into the magnetization reversal process in oxide-based junctions, which here strongly limits the TMR. Inducing uniaxial anisotropy, for instance by growing the films on (100)-oriented orthorhombic substrates such as NdGaO 3 (ref. 51 ), could be beneficial. We have also addressed the role of the interface-induced magnetic state on spin-dependent transport. Due to the antiparallel alignment of the induced moment in LFO with that in LSMO, the exchange splitting in the barrier results in spin-filtering effects that favour the transmission of spin-down carriers. They thus tend to reduce or even reverse the (initially positive) spin-polarization of electrons tunnelling from LSMO. These spin-filtering effects manifest mainly in two ways: they strongly decrease the TMR in the ferromagnetic regime of the barrier and they produce a nonmonotonous bias dependence of the TMR, that first rises with bias, shows a maximum and then decreases. An important contribution of this research is the use of the spintronic response of MTJs to probe the magnetic and electronic states of correlated oxide interfaces. An extension of this work could be to explore other barrier materials in which the induced magnetic moment would be parallel to that in the electrode, thus summing the spin-filtering effect with the conventional tunnelling magnetoresistance. This would result in an enhanced TMR at low and high bias voltages, reducing the detrimental influence of inelastic spin-depolarizing mechanisms. The semi-empirical Goodenough–Kanamori–Anderson rules of super-exchange predict that this may be achieved in several systems, for instance, combining manganites and nickelates. For room-temperature operation, transition metal electrodes may, however, be necessary. The recent detection of magnetic moments generated in nonmagnetic perovskites at the interface with ferromagnetic metals [52] suggests that the interface-induced spin-filtering effects that we have described here may also be found at room temperature and above. Sample growth Samples were grown in a high pressure pure oxygen sputtering system. This method produces oxide layers with good epitaxial properties. The growth temperature was set to 800 °C. Oxygen pressure during growth was P O2 =2.8 mbar. After the deposition, the samples were annealed during 10 min at 750 °C under an oxygen pressure of 900 mbar before cooling down at a rate of 20 °C min −1 . X-ray reflectivity XRR was performed in a four-circle Philips Xpert-PRO MRD diffractometer with Cu cathode (wavelength λ =0.15418, nm). Magnetometry Magnetic characterization of single films and of LFO/LSMO and LSMO/LFO bilayers was performed with SQUID and VSM magnetometers installed in a PPMS (Quantum Design) apparatus in a temperature range 1.7–400 K and in variable magnetic fields (up to 14 T). STEM–EELS Electron microscopy observations were carried out in an aberration-corrected Nion UltraSTEM100 operated at 100 kV and equipped with a Gatan Enfina EEL spectrometer. To obtain the EELS maps, principal component analysis was used to remove random noise and the intensities under the edges were integrated after background subtraction using a power law. Samples were prepared using conventional methods, grinding and Ar ion milling. Element selective chemical and magnetic characterization X-ray absorption spectra were measured by means of fluorescence yield detection. The incoming circular-polarized radiation impinged the sample at a gracing incidence angle of 10 degrees. The data were obtained as a function of temperature across the Mn and Fe L 3,2 edges in magnetic remanence after saturating the in-plane magnetization for both positive and negative fields. This set up optimizes the signal-to-noise ratio for the XMCD, that is, calculated as the difference between the XAS curves obtained for positive and negative fields. The XAS spectra are obtained by averaging the XAS spectra for positive and negative fields, thus removing the magnetic contribution. Element selective magnetic hysteresis loops were measured at the Mn and Fe L 3 edges by means of XMCD in reflection geometry, that is, X-ray resonant magnetic scattering. Scattering was measured in a theta/2-theta geometry as a function of the in-plane magnetic field for incoming circular-polarized light. PEEM For magnetic imaging, the photon energy was tuned to the L 3 resonance of iron or manganese, exploiting the element-specific XMCD. Each of the XMCD images shown was calculated from a sequence of images taken with circular polarization (90% of circular photon polarization) and alternating helicity. After normalization to a bright-field image, the sequence was drift-corrected, and frames were recorded at the same photon energy and polarization have been averaged. The magnetic contrast is shown as the difference of the two average images with opposite helicity, divided by their sum. The magnetic contrast represents the magnetization component pointing along the incidence direction of the X-ray beam. An in-plane magnetic field was applied in situ to the films during data acquisition by a coil attached to the sample holder. Lithography Selected LSMO/LFO/LSMO trilayers were patterned into tunnel junctions using a combination of optical lithography, ion-beam etching, reactive ion etching and lift off, following ref. 37 . Transport measurement Transport measurements were performed in a continuous He flow cryostat after cooling down the sample with no magnetic field applied (zero-field cooling). Subsequent I(V) and R(H) data were obtained at different temperatures in four-wire configuration by applying a fixed direct current (dc) bias voltage and measuring current. Transport simulations We perform the simulation using a numerical model based on WKB approximation. In WKB approximations, the transmission probability T for an electron with energy E can be expressed as follows in atomic units: Here φ B is the barrier height (taken to be 0.252 eV); σ and σ′ are the spin directions (up or down) of the electrons in the left and right electrode, respectively. Near the interfaces where the LFO develops a ferromagnetic-like moment, the barrier potential profile is exchange splitted. Because the moment in LFO is antiparallel to that in LSMO, we assume that the barrier height for spin-up carriers is higher than that for spin down. The potential profile can thus be described as follows. In the parallel configuration, we have: and in the antiparallel configuration: with Δ ex =0.192 eV. We suppose that the LFO barrier is ferromagnetic like over three unit cells at each interface, that is x left = t − x right =1.2 nm. Finally, the Fowler–Nordheim regime was modelled by assuming a voltage-dependent barrier length in the WKB approximation at first order. In our calculation, we neglect all interferences or scattering events and also do not calculate the real part of the tunnelling electrons’ wave vectors that do not contribute to the decay probability. To account for the total dc conductance under finite biases, we performed integration over all the available states when the Fermi level of one electrode is raised above that of the other. Mathematically, the total dc conductance G at bias voltage V is expressed as follows, Here f ( E ) is the Fermi distribution function and N σ , N σ ′ are the density of states (DOS) of the electrodes on the two sides. For simplicity, we assume that the LSMO electrode has flat DOS regarding the relatively small voltage range we are exploring and that the electric field is homogeneous throughout the barrier. The TMR ratio is thus simply TMR=( G p − G ap )/ G ap with G ap (respectively G p ) being calculated for σ ≠ σ ′ (respectively σ = σ ′). Considering the large energies involved in the problem compared with thermal activation, we computed the above formula at 0 K, which results in a finite integral from 0 to –eV. The integral on x was calculated analytically and the one on voltage by numerical summation over a mesh of V /1,000 in voltage. Finally, all the inelastic effects that are necessary to model the behaviour at 100 K are modelled in both cases by a Lorentzian decay such that , with V 1/2 =0.126 V at T =100 K and V 1/2 =0.03 V at T =50 K. We take a low-temperature spin polarization of 0.93 for both LSMO electrodes. How to cite this article: Bruno, F. Y. et al. Insight into spin transport in oxide heterostructures from interface-resolved magnetic mapping. Nat. Commun. 6:6306 doi: 10.1038/ncomms7306 (2015).